αB-crystallin interacts with and prevents stress-activated proteolysis of focal adhesion kinase by calpain in cardiomyocytes Focal adhesion kinase (FAK) contributes to cellular homeostasis under stress conditions. Here we show that αB-crystallin interacts with and confers protection to FAK against calpain-mediated proteolysis in cardiomyocytes. A hydrophobic patch mapped between helices 1 and 4 of the FAK FAT domain was found to bind to the β4–β8 groove of αB-crystallin. Such an interaction requires FAK tyrosine 925 and is enhanced following its phosphorylation by Src, which occurs upon FAK stimulation. αB-crystallin silencing results in calpain-dependent FAK depletion and in the increased apoptosis of cardiomyocytes in response to mechanical stress. FAK overexpression protects cardiomyocytes depleted of αB-crystallin against the stretch-induced apoptosis. Consistently, load-induced apoptosis is blunted in the hearts from cardiac-specific FAK transgenic mice transiently depleted of αB-crystallin by RNA interference. These studies define a role for αB-crystallin in controlling FAK function and cardiomyocyte survival through the prevention of calpain-mediated degradation of FAK. Exposure to stress increases the risk of intracellular protein unfolding and aggregation, thus compromising cell viability. To reduce this danger, cells rely on an elaborate arsenal of molecular chaperones and clearance mechanisms that utilize proteolytic systems, which act to maintain protein homeostasis [1] . The failure of these systems is emerging as a major mechanism underlying several pathological conditions, such as cancer, neurodegenerative and cardiovascular diseases [2] , [3] . Among protein chaperones, the small heat–shock proteins (sHSPs, ranging from 12 to 42 kDa) have unique capacities to bind and prevent the aggregation of partially unfolded proteins under conditions of cellular stress [4] . sHSPs share a conserved α-crystallin domain (ACD), a sequence of seven to eight beta strands that are flanked by a diverse amino-terminal arm and a moderately conserved carboxy-terminal extension. The ACD is essential for the assembly of dimers and higher-order oligomers, but it is also required for the function of sHSPs [5] , [6] , [7] . The prototypical sHSP, αB-crystallin (22 kDa), is constitutively expressed in the eye lens and in several other tissues, notably, the cardiac and skeletal muscles and the brain [4] . In muscles, αB-crystallin binds to intermediate filaments and sarcomeric myofibrils, preventing their irreversible aggregation during stress [8] , [9] . It is therefore not surprising that inherited defects and the experimental gene targeting of αB-crystallin result in protein deposition diseases of cardiac and skeletal muscles [10] , [11] . However, in addition to its primordial duty as a molecular chaperone, αB-crystallin plays critical roles in essential cellular processes, including differentiation and survival [12] , [13] , suggesting that it may function as a key component in signal transduction networks. Accordingly, αB-crystallin is known to bind and modulate the activity of several signalling proteins in their native state, including Bax, Bcl-2 and p53 (refs 14 , 15 ); the knowledge of this regulation is rapidly emerging. Focal adhesion kinase (FAK) is a mediator of the hypertrophic growth and survival of cardiomyocytes during mechanical stress [16] , [17] , [18] , [19] . However, the regulation of FAK in this particular cell type remains unclear. One current model suggests that following its activation, FAK Y397 becomes autophosphorylated, creating a binding site for Src, which then phosphorylates other tyrosine residues of the catalytic and the C-terminal FAK domains [20] . The phosphotyrosines function to enhance FAK catalytic activity and to activate downstream signalling molecules and scaffolding proteins [21] , [22] . In particular, the Src-dependent phosphorylation of Y925 is linked to the regulation of FAK subcellular localization and downstream signalling by ERK1/2 (refs 22 , 23 ). Furthermore, the level of FAK activity can be regulated by calpain-mediated proteolysis. In fact, this method seems to be a mechanism for inhibiting FAK activity at focal adhesions, which is required to promote cell migration [24] . Since both FAK and αB-crystallin play active roles in modulating cellular response to stress, we investigated whether they mechanistically integrate into a signalling pathway. We found that mechanical stress triggers a functionally important interaction of FAK with αB-crystallin in cardiomyocytes. A combination of structural, imaging and biochemical tools was used to determine that the FAK’s C-terminal focal adhesion-targeting (FAT) domain mediates its interaction with αB-crystallin. Through this interaction, FAK is protected from degradation by calpain and contributes to reduce the cardiomyocyte susceptibility to apoptosis during mechanical stress. Thus, the recruitment of FAK by αB-crystallin meets independent requirements for the regulation of FAK signalling and impacts the ability of cardiomyocytes to cope with mechanical stress. FAK associates with αB-crystallin in response to stress To determine whether αB-crystallin interacts with FAK during mechanical stress, we initially studied ventricular cardiomyocytes derived from 2-day-old neonatal rats (neonatal rat ventricular myocytes (NRVMs)) cultured on a silicone-based membrane system. The controlled biaxial cyclic stretch (10% from the slack length; 60 Hz; 1–12 h) of the NRVMs increased the FAK Y397 phosphorylation ( Fig. 1a ), which is a hallmark of FAK activation and functions in Src recruitment and activation [20] . FAK Y925 phosphorylation, which has been recognized as an Src-dependent process [22] , was also enhanced in stretched cells ( Fig. 1a ). No obvious change in the FAK protein level was noticed in the stretched compared with the non-stretched cultures. A parallel immunoblot analysis revealed increases in the levels of αB-crystallin protein and chaperone-activating S59 phosphorylation in the stretched versus non-stretched NRVMs ( Fig. 1a ). To evaluate a potential interaction between FAK and αB-crystallin, we immunoprecipitated NRVM extracts with an anti-αB-crystallin antibody. An association between FAK and αB-crystallin was detected in the extracts of stretched, whereas only a minor association was expressed in the extracts of the non-stretched NRVMs ( Fig. 1b ). The ratio between the amounts of FAK and αB-crystallin precipitated by the anti-αB-crystallin antibody following cell stretch increased up to twofold over the non-stretched controls ( Fig. 1b ). Furthermore, the αB-crystallin immunoprecipitates obtained from the stretched cells were enriched with Y397- and Y925-phosphorylated FAK, suggesting that αB-crystallin associates with the active form of FAK ( Fig. 1c,d ). Changes in FAK and αB-crystallin in NRVMs were further evaluated by immunocytochemistry. In non-stretched myocytes, the distribution of FAK was sarcomeric and cytoplasmic, concentrated in the perinuclear region, while αB-crystallin displayed a perinuclear distribution, with no obvious association with the sarcomeres ( Fig. 1e ). In these cells, perinuclear FAK and αB-crystallin barely overlapped in merged images. Cell stretch enhanced αB-crystallin signal and induced its localization to the sarcomeres, where it overlaps with FAK ( Fig. 1e ). 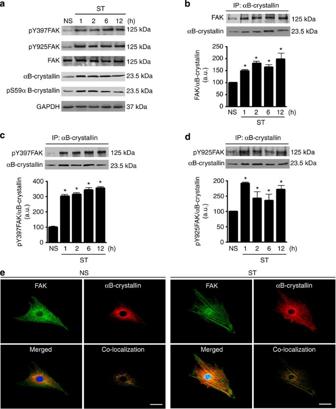Figure 1: FAK interacts with αB-crystallin in cardiomyocytes. (a) Representative immunoblots of six independent experiments showing extracts from NS or ST (1, 2, 6 and 12 h) NRVMs probed as indicated. GAPDH served as loading control. (b–d) Representative (n=6) anti-FAK, -pY397-FAK and anti-pY925-FAK immunoblots of αB-crystallin immunoprecipitates (IP) from extracts of NS or ST NRVMs (1, 2, 6 and 12 h). Bar graphs show the densitometric readings of FAK, pY397-FAK and pY925-FAK normalized to αB-crystallin. *P<0.0001 versus NS NRVMs (Pvalues were determined by analysis of variance and Bonferroni’spost hoccomparisons). Data are presented as mean±s.e.m. (e) Confocal immunofluorescence imaging of NS or ST (2 h) NRVMs stained with anti-FAK and anti-αB-crystallin. FAK distribution is shown in green and αB-crystallin is shown in red. Merged images are composed of anti-FAK, anti-αB-crystallin and DAPI stained. Regions of co-localization are shown as separate images. Scale bar, 20 μm. IP, immunoprecipitation; NS, non-stretched; ST, stretched. Figure 1: FAK interacts with αB-crystallin in cardiomyocytes. ( a ) Representative immunoblots of six independent experiments showing extracts from NS or ST (1, 2, 6 and 12 h) NRVMs probed as indicated. GAPDH served as loading control. ( b – d ) Representative ( n =6) anti-FAK, -pY397-FAK and anti-pY925-FAK immunoblots of αB-crystallin immunoprecipitates (IP) from extracts of NS or ST NRVMs (1, 2, 6 and 12 h). Bar graphs show the densitometric readings of FAK, pY397-FAK and pY925-FAK normalized to αB-crystallin. * P <0.0001 versus NS NRVMs ( P values were determined by analysis of variance and Bonferroni’s post hoc comparisons). Data are presented as mean±s.e.m. ( e ) Confocal immunofluorescence imaging of NS or ST (2 h) NRVMs stained with anti-FAK and anti-αB-crystallin. FAK distribution is shown in green and αB-crystallin is shown in red. Merged images are composed of anti-FAK, anti-αB-crystallin and DAPI stained. Regions of co-localization are shown as separate images. Scale bar, 20 μm. IP, immunoprecipitation; NS, non-stretched; ST, stretched. Full size image To investigate whether the association between FAK and αB-crystallin occurs in response to distinct forms of cellular stress, we treated H9c2 cardiac myoblasts with hydrogen peroxide (H 2 O 2 ). After the treatment with H 2 O 2 (1 mM, 10–120 min), the abundance of αB-crystallin and Y397-phosphorylated FAK were significantly increased ( Supplementary Fig. 1a ). Treatment with H 2 O 2 also markedly enhanced the association of FAK with αB-crystallin in H9c2 cells, expressed by the ratio between the amounts of FAK and αB-crystallin precipitated by the anti-FAK antibody ( Supplementary Fig. 1b ). We then examined FAK and αB-crystallin distribution in H9c2 cells. In untreated cells, FAK localizes prominently to adhesions and less intensely along the stress fibres and in the perinuclear region, while αB-crystallin distributes in the cytoplasm, concentrated at the perinuclear region ( Supplementary Fig. 1c ). In these cells, FAK co-localizes with αB-crystallin in the perinuclear region, but not at focal adhesions. Cells treated with H 2 O 2 reveal no substantial change in FAK localization, but show an increase in the cytoplasmic αB-crystallin, which corresponds to the increased expression detected in the western blots. Consistent with the results of co-immunoprecipitation assays, FAK and αB-crystallin co-localization increases in cells treated with H 2 O 2 , mainly in the cytoplasm and along the stress fibres ( Supplementary Fig. 1c ). Because αB-crystallin translocates to mitochondria under stress conditions [25] , we investigated whether the FAK-αB-crystallin complexes formed in response to oxidative stress in H9c2 are localized in mitochondria. Cells were probed with anti-FAK and anti-αB-crystallin antibodies and the mitochondria marker Mitotracker ( Supplementary Fig. 1d ). In cells treated with H 2 O 2 , αB-crystallin partially co-localized with mitochondria, but FAK did not, indicating that the fraction of αB-crystallin bound to FAK in stressed cells is not associated with mitochondria. FAK associates with αB-crystallin in overloaded rat heart To explore whether the association between FAK and αB-crystallin occurs under acute pathophysiological conditions in adult hearts, we examined samples of rat left ventricle subjected to 2 h of pressure overload induced by transverse aortic constriction (TAC). FAK phosphorylation at Y397 and Y925 were increased, while the FAK protein levels remained unaltered in this model ( Fig. 2a ). Acute pressure overloading also increased the levels of αB-crystallin protein and Ser-59 phosphorylation and the association with FAK in the rat left ventricle ( Fig. 2a ). The ratio between the amounts of FAK and αB-crystallin precipitated by the anti-αB-crystallin antibody increased twofold in the overloaded over the left ventricle of sham-operated (SO) mice ( Supplementary Fig. 2a ). Additional analyses demonstrated increased levels of Y397- and Y925-phosphorylated FAK in the anti-αB-crystallin precipitates obtained from the lysates of the overloaded left ventricle ( Fig. 2a ). We also demonstrated that FAK phosphorylation, αB-crystallin expression and FAK association with αB-crystallin were increased in adult cardiomyocytes isolated from overloaded rat left ventricle compared with those isolated from control rats ( Fig. 2b ; Supplementary Fig. 2b ). Furthermore, immunohistochemistry of the rat left ventricle revealed an enhanced co-localization of FAK and αB-crystallin at the sarcomeres of cardiomyocytes from overloaded compared with the control hearts ( Fig. 2c ). Collectively, these results indicate that FAK associates with αB-crystallin in cardiomyocytes. This association accompanies FAK activation, suggesting that αB-crystallin may participate in the regulation of FAK signalling in cardiomyocytes and in the heart of rat. 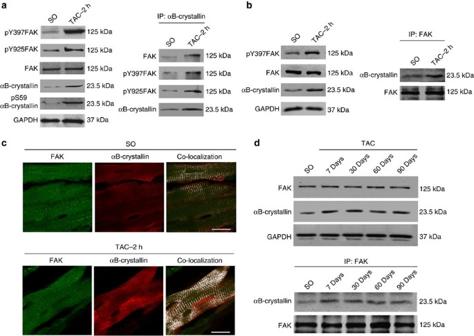Figure 2: Mechanical stress increases the association of FAK with αB-crystallin in overloaded left ventricle of rodents. (a) Representative western blots of anti-FAK, -pY397-FAK, -pY925FAK, -αB-crystallin, -p59αB-crystallin and -GAPDH antibodies obtained with extracts of the left ventricle from SO (n=6) or TAC (2 h;n=6) rats. GAPDH served as loading control; at right, anti-FAK, -pY397-FAK and anti-pY925-FAK immunoblots of anti-αB-crystallin immunoprecipitates (IP). αB-crystallin was used as loading control. (b) Shown are specific immunoblots of extracts from isolated adult cardiomyocytes obtained from SO (n=4) or TAC (2 h;n=4) rats, as indicated. Representative anti-αB-crystallin and -FAK immunoblots of anti-FAK immunoprecipitates (IP) are shown on the right. FAK was used as loading control. (c) Confocal imaging of anti-FAK and anti-αB-crystallin double-labelled ventricular tissue from SO and TAC (2 h) rats. FAK distribution is shown in green and αB-crystallin is shown in red. Regions of co-localization between anti-FAK and anti-αB-crystallin stainings are indicated in white. Scale bar, 20 μm. (d) Representative western blottings showing FAK, αB-crystallin and GAPDH expression in samples of the left ventricle from SO (n=5) or TAC (7, 30, 60 and 90 days;n=5 for each group) mice. GAPDH served as loading control. Lower panel shows representative anti-αB-crystallin and anti-FAK immunoblottings of the anti-FAK immunoprecipitated from extracts of left ventricle from SO and TAC mice. FAK served as loading control. IP, immunoprecipitation. Figure 2: Mechanical stress increases the association of FAK with αB-crystallin in overloaded left ventricle of rodents. ( a ) Representative western blots of anti-FAK, -pY397-FAK, -pY925FAK, -αB-crystallin, -p59αB-crystallin and -GAPDH antibodies obtained with extracts of the left ventricle from SO ( n =6) or TAC (2 h; n =6) rats. GAPDH served as loading control; at right, anti-FAK, -pY397-FAK and anti-pY925-FAK immunoblots of anti-αB-crystallin immunoprecipitates (IP). αB-crystallin was used as loading control. ( b ) Shown are specific immunoblots of extracts from isolated adult cardiomyocytes obtained from SO ( n =4) or TAC (2 h; n =4) rats, as indicated. Representative anti-αB-crystallin and -FAK immunoblots of anti-FAK immunoprecipitates (IP) are shown on the right. FAK was used as loading control. ( c ) Confocal imaging of anti-FAK and anti-αB-crystallin double-labelled ventricular tissue from SO and TAC (2 h) rats. FAK distribution is shown in green and αB-crystallin is shown in red. Regions of co-localization between anti-FAK and anti-αB-crystallin stainings are indicated in white. Scale bar, 20 μm. ( d ) Representative western blottings showing FAK, αB-crystallin and GAPDH expression in samples of the left ventricle from SO ( n =5) or TAC (7, 30, 60 and 90 days; n =5 for each group) mice. GAPDH served as loading control. Lower panel shows representative anti-αB-crystallin and anti-FAK immunoblottings of the anti-FAK immunoprecipitated from extracts of left ventricle from SO and TAC mice. FAK served as loading control. IP, immunoprecipitation. Full size image We next examined whether the association between FAK and αB-crystallin in cardiomyocytes persists during the transition of compensated to decompensated hypertrophy. Mice were subjected to 7–90-day TAC, which results in concentric hypertrophy of the left ventricle by 7 days, followed by progressive left ventricular dilation thereafter, as confirmed by M-mode echocardiography (see Supplementary Table 1 ). Importantly, FAK expression in the left ventricle did not change in response to TAC. However, the expression of αB-crystallin and its association with FAK, as detected in the immunoprecipitates of anti-FAK antibody, increased (twofold) early and remained increased throughout the observational period ( Fig. 2d ; Supplementary Fig. 2c ). These data suggest that the association between FAK and αB-crystallin may have an important role in controlling FAK signalling and cardiac homeostasis in pathophysiological conditions. αB-crystallin interacts directly with the C terminus of FAK To determine whether αB-crystallin can bind FAK directly, we performed pull-down assays using recombinant glutathione S-transferase (GST)-tagged full-length FAK (GST-FAK; Invitrogen) and 6xHis-tagged αB-crystallin (His-CryAB) proteins. His-CryAB was expressed in Escherichia coli and purified to homogeneity by affinity and size-exclusion chromatography (SEC; Supplementary Fig. 3a ). Unlike the GST control, GST-FAK interacted with His-CryAB ( Fig. 3a ). In separate studies, His-CryAB was shown to precipitate greater amounts of FAK from extracts of stretched NRVMs compared with non-stretched NRVMs ( Fig. 3b ). Next, recombinant GST-fusion proteins that covered the N-terminal FERM (GST-FERM), the kinase (GST-Kinase) and the C-terminal (GST-cTERM) domains of FAK were expressed in E. coli and purified to homogeneity ( Supplementary Fig. 3b ). These constructions were coupled to glutathione sepharose beads and assayed for binding to His-CryAB. The GST-cTERM was the only construct that interacted with His-CryAB, indicating that this domain is sufficient to confer FAK interaction with αB-crystallin ( Fig. 3c ). Likewise, FAK GST-cTERM was the only construct that precipitated αB-crystallin from NRVM extracts ( Fig. 3d ). Consistent with the co-immunoprecipitation data, the amount of αB-crystallin precipitated by the GST-cTERM construct increased when samples of stretched (rather than non-stretched) myocytes were used. 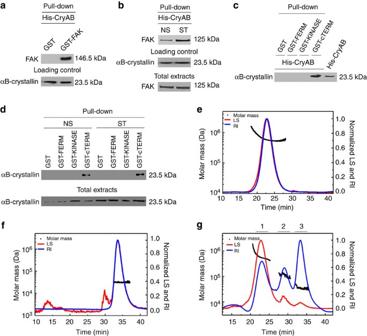Figure 3: FAK C terminus mediates the direct interaction of FAK with αB-crystallin. (a) Representative (n=4) anti-FAK immunoblot from His pull-down assay of FAK (GST-FAK) performed with His-CryAB coupled to Ni2+Sepharose beads. GST alone was used as negative control. Anti-αB-crystallin immunoblots were used as loading control. (b) Representative (n=4) anti-FAK immunoblot from pull-down assays of extracts from NS or ST (2 h) NRVMs performed with His-CryAB. αB-crystallin was used as loading control. Amounts of FAK in the extracts of the NS or ST NRVMs were analysed by immunoblotting probed with anti-FAK. (c) Representative (n=4) αB-crystallin immunoblot from pull-down assay of His-CryAB performed with recombinant FAK fragments (GST-FERM, GST-Kinase or GST-cTERM) and GST alone as control. (d) Representative (n=4) anti-αB-crystallin immunoblot from pull-down assays of extracts from NS or ST NRVMs performed with recombinant FAK fragments (GST-FERM, GST-Kinase or GST-cTERM) and GST alone (upper panel). The lower immunoblot shows the amount of αB-crystallin from NS or ST NRVM total extracts. (e) The SEC-MALS chromatograms show the refractive index (blue line), light-scattering (red line) intensity (90° detector) and calculated molar mass (black squares). His-CryAB elutes as a single peak centred on a maximum population species of 580 kDa, corresponding to an ~28-subunit oligomer. (f) SEC-MALS shows His-FAK-cTERM eluting as a single peak of 32±1 kDa, in agreement with the monomer molar mass. (g) SEC-MALS profile of His-CryAB and His-cTERM mixture. His-CryAB and His-cTERM interaction resulted in shifts in the retention time and molecular weight from the individual components. The complex formed by His-CryAB and His-FAK-cTERM eluted between the peaks of isolated proteins, with an average molar mass of 114±1 kDa, in agreement with a 2:2 stoichiometry. The SEC-MALS assays were carried out on a GE Healthcare Superdex200 HR 10/30 column connected to the multi-angle laser light-scattering system and are representative of six independent experiments. Figure 3: FAK C terminus mediates the direct interaction of FAK with αB-crystallin. ( a ) Representative ( n =4) anti-FAK immunoblot from His pull-down assay of FAK (GST-FAK) performed with His-CryAB coupled to Ni 2+ Sepharose beads. GST alone was used as negative control. Anti-αB-crystallin immunoblots were used as loading control. ( b ) Representative ( n =4) anti-FAK immunoblot from pull-down assays of extracts from NS or ST (2 h) NRVMs performed with His-CryAB. αB-crystallin was used as loading control. Amounts of FAK in the extracts of the NS or ST NRVMs were analysed by immunoblotting probed with anti-FAK. ( c ) Representative ( n =4) αB-crystallin immunoblot from pull-down assay of His-CryAB performed with recombinant FAK fragments (GST-FERM, GST-Kinase or GST-cTERM) and GST alone as control. ( d ) Representative ( n =4) anti-αB-crystallin immunoblot from pull-down assays of extracts from NS or ST NRVMs performed with recombinant FAK fragments (GST-FERM, GST-Kinase or GST-cTERM) and GST alone (upper panel). The lower immunoblot shows the amount of αB-crystallin from NS or ST NRVM total extracts. ( e ) The SEC-MALS chromatograms show the refractive index (blue line), light-scattering (red line) intensity (90° detector) and calculated molar mass (black squares). His-CryAB elutes as a single peak centred on a maximum population species of 580 kDa, corresponding to an ~28-subunit oligomer. ( f ) SEC-MALS shows His-FAK-cTERM eluting as a single peak of 32±1 kDa, in agreement with the monomer molar mass. ( g ) SEC-MALS profile of His-CryAB and His-cTERM mixture. His-CryAB and His-cTERM interaction resulted in shifts in the retention time and molecular weight from the individual components. The complex formed by His-CryAB and His-FAK-cTERM eluted between the peaks of isolated proteins, with an average molar mass of 114±1 kDa, in agreement with a 2:2 stoichiometry. The SEC-MALS assays were carried out on a GE Healthcare Superdex200 HR 10/30 column connected to the multi-angle laser light-scattering system and are representative of six independent experiments. Full size image To gain information about the stoichiometry of FAK-cTERM and αB-crystallin assembly, we used recombinant His-CryAB and FAK His-cTERM ( Supplementary Fig. 3c ) and SEC coupled to a multi-angle light-scattering (MALS) detector. First, we investigated the mass distribution of the His-CryAB oligomer at room temperature. The protein eluted from the column as a single broad, but slightly asymmetric, peak centred on ~22.7 min ( Fig. 3e ). The MALS data shows that at the front end of the peak, the average mass was ~750 kDa, at the tail end 550 kDa and at the maximum 580 kDa. This corresponds to an approximate average-oligomer distribution range of 24–32 subunits. His-cTERM was also characterized by SEC-MALS, and it was shown to be a monomer in solution ( Fig. 3f ). The protein eluted from the column as a single peak with average mass of 32±1 kDa centred on ~33.5 min. The SEC-MALS approach of the samples containing the complex His-cTERM-His-CryAB showed three distinct peaks. The first one corresponds to the His-CryAB elution, the late one corresponds to His-cTERM elution and the middle peak (centred on ~29 min) corresponds to the complex His-cTERM-His-CryAB elution ( Fig. 3g ; Supplementary Fig. 3d ). The MALS data from the maximum of the middle peak correspond to an average mass of ~114±1 kDa. Theoretically, this mass corresponds to a 2:2 stoichiometry of His-CryAB (~23 kDa) and FAK-cTERM (~34 kDa). This stoichiometry was confirmed by experiments where the His-cTERM/His-CryAB complex peak was isolated by SEC and re-examined by SEC-MALS ( Supplementary Fig. 3e ). Collectively, these results indicate that FAK binds to the chaperone αB-crystallin through a direct interaction that is mediated by its C-terminal domain. The ability of His-CryAB to act as a molecular chaperone was assessed via its capacity to prevent the aggregation of FAK-cTERM denatured by heat. FAK His-cTERM was incubated at 42 °C in the presence or absence of His-CryAB at molar ratio (His-CryAB:FAK-cTERM) of 1:1. The precipitated and soluble proteins were separated by centrifugation and resolved by SDS–polyacrylamide gel electrophoresis (SDS-PAGE). FAK His-cTERM was precipitated in the absence, but not in the presence of His-CryAB, indicating that this construct of αB-crystallin retains its chaperone activity ( Supplementary Fig. 4 ). FAK-cTERM-αB-crystallin interaction in living cells To determine whether FAK-cTERM interacts with αB-crystallin in living cells, we employed an assay to detect FAK-cTERM-αB-crystallin proximity by Förster resonance energy transfer (FRET) in HEK 293T cells. In this assay, the cyan fluorescent protein (CFP) coupled to the N terminus of αB-crystallin (CFP-CryAB) served as the FRET donor, while the yellow fluorescent protein (YFP) coupled to the N terminus of FAK-cTERM (YFP-cTERM) served as the FRET acceptor ( Supplementary Fig. 5 ). In our system, only the constructs that have the fluorescent proteins (CFP and YFP) fused to the N terminus of αB-crystallin and FAK-cTERM resulted in efficient FRET. FRET was measured here using fluorescence lifetime imaging microscopy (FLIM). If energy transfer occurs, the lifetime of the donor-emitted fluorescence will decrease because of the new decay path. Plasmid vectors encoding unfused CFP and YFP were co-transfected in cells as negative controls. Despite the co-localization of the donor–acceptor fluorophores in the confocal images, the fluorescence lifetime-weighted mean component ( τ m ) of the donor was 2.5 ns, indicating the absence of FRET ( Fig. 4a ). A highly efficient positive FRET control was obtained with the CFP fluorophore that was coupled directly to YFP through a 15-amino-acid (aa)-long linker ( Fig. 4b ). The lifetime of CFP decreased to 1 ns, indicating the proximity of CFP to YFP. The τ m of CFP-CryAB co-expressed with YFP was 2.4 ns ( Fig. 4c ), while the co-expression of the pair CFP-CryAB and YFP-cTERM decreased the donor lifetime to 1.8 ns ( Fig. 4d ). No major difference was observed in the distribution of CFP-CryAB and YFP-cTERM in cells co-expressing both constructs compared with cells expressing each of the constructs alone ( Fig. 4d ; Supplementary Fig. 5 ). The reduction in the lifetime of the CFP-CryAB confirmed a positive FRET between CFP-CryAB and YFP-cTERM. Thus, the FRET assay data support a direct interaction between FAK-cTERM and αB-crystallin in living cells. 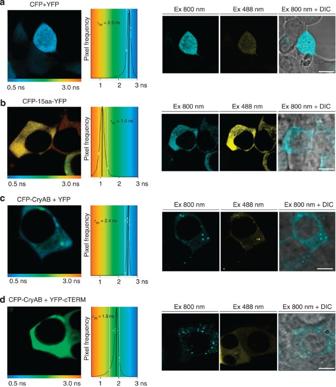Figure 4: Confocal imaging of cells transfected with the donor and acceptor FRET pair. (a,b) Lifetime images of HEK 293T cells transfected withpAmCyan1-C1andpZsYellow1-C1vectors (negative control) or with thepAmCyan1-C1encoding the YFP linked to CFP through a 15-aa-long linker (positive control). In this positive control, the fluorescence lifetime,τm, of the donor (2.5 ns) was reduced to 1.0 ns. (c,d) Lifetime images of HEK 293T cells transfected withpAmCyan1-C1-CryABpluspZsYellow1-C1 vectorsor with thepAmCyan1-C1-CryABpluspZsYellow1-C1-cTERMvectors. The fluorescence lifetime of the donor CFP-CryAB (2.4 ns) was reduced to 1.8 ns by FRET. The correspondent images representing the fluorescence (excitation at 800 and 488 nm) and differential interference contrast microscopy (DIC) of cells are displayed at the right panels. Scale bar, 10 μm. Figure 4: Confocal imaging of cells transfected with the donor and acceptor FRET pair. ( a , b ) Lifetime images of HEK 293T cells transfected with pAmCyan1-C1 and pZsYellow1-C1 vectors (negative control) or with the pAmCyan1-C1 encoding the YFP linked to CFP through a 15-aa-long linker (positive control). In this positive control, the fluorescence lifetime, τ m , of the donor (2.5 ns) was reduced to 1.0 ns. ( c , d ) Lifetime images of HEK 293T cells transfected with pAmCyan1-C1-CryAB plus pZsYellow1-C1 vectors or with the pAmCyan1-C1-CryAB plus pZsYellow1-C1-cTERM vectors. The fluorescence lifetime of the donor CFP-CryAB (2.4 ns) was reduced to 1.8 ns by FRET. The correspondent images representing the fluorescence (excitation at 800 and 488 nm) and differential interference contrast microscopy (DIC) of cells are displayed at the right panels. Scale bar, 10 μm. Full size image Y925 phosphorylation enhances FAK-αB-crystallin interaction We next asked whether the phosphorylation of FAK-cTERM at Y925 could influence the interaction with αB-crystallin. To test this hypothesis, we performed pull-down assays with a recombinant GST-tagged αB-crystallin (GST-CryAB) coupled to glutathione sepharose beads, and His-FAK-cTERM, Y925-phosphorylated His-FAK-cTERM and a Y925F mutant His-FAK-cTERM. The Y925-phosphorylated FAK-cTERM was obtained by performing in vitro phosphorylation with Src ( Fig. 5a ; Supplementary Fig. 6a ). This phosphorylation was confirmed by immunoblot with a phosphospecific antibody and by tandem mass spectrometry (MS/MS) analysis ( Supplementary Fig. 6b,c ). Y925 phosphorylation markedly enhanced the binding of FAK-cTERM to GST-CryAB, whereas the cTERM mutation Y925F abolished the interaction ( Fig. 5b ). The MALS data of cTERM-Y925F showed no change in its elution pattern with respect to cTERM-WT ( Fig. 5c ), but the co-elution with His-CryAB (peak centred on ~29 min) was disrupted ( Fig. 5d ). These results indicate that Y925 is required for the interaction of FAK-cTERM with αB-crystallin and that its phosphorylation by Src enhances this interaction. 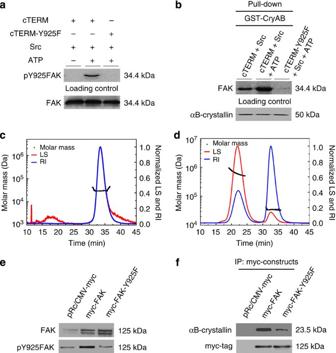Figure 5: Tyr925 phosphorylation enhances FAK-αB-crystallin interaction. (a)In vitroSrc kinase assay performed with FAK-cTERM, FAK-cTERM-Y925F, recombinant Src kinase and ATP, as indicated. Shown are immunoblots performed with anti-pY925-FAK and anti-FAK antibodies. Immunoblottings performed with anti-FAK were used as loading control. (b) FAK immunoblot from GST-CryAB pull-down assay of FAK His-cTERM, FAK His-cTERM-Y925F, recombinant Src kinase and ATP performed as indicated. αB-crystallin immunoblots were used as loading control (n=4 independent experiments). (c) SEC-MALS chromatogram of His-FAK-cTERM-Y925F shows its elution as a single peak of 32±1 kDa. (d) SEC-MALS profile of His-CryAB and His-cTERM-Y925F mixture. His-CryAB and His-cTERM-Y925F elute as isolated proteins. The first peak corresponds to His-CryAB (600±5 kDa) and the second to His-cTERM-Y925F (34±1 kDa). (e) FAK and pY925-FAK immunoblots of protein extracts from C2C12 cells transfected withpRc/CMV-myc,pRc/CMV-myc-FAK(myc-FAK) orpRc/CMV-myc-FAK-Y925F(myc-FAK-Y925F) vectors. (f) Representative (n=4) anti-αB-crystallin and anti-myc-tag immunoblots of anti-myc-tag immunoprecipitates (IP) from C2C12 cells treated as indicated. Figure 5: Tyr925 phosphorylation enhances FAK-αB-crystallin interaction. ( a ) In vitro Src kinase assay performed with FAK-cTERM, FAK-cTERM-Y925F, recombinant Src kinase and ATP, as indicated. Shown are immunoblots performed with anti-pY925-FAK and anti-FAK antibodies. Immunoblottings performed with anti-FAK were used as loading control. ( b ) FAK immunoblot from GST-CryAB pull-down assay of FAK His-cTERM, FAK His-cTERM-Y925F, recombinant Src kinase and ATP performed as indicated. αB-crystallin immunoblots were used as loading control ( n =4 independent experiments). ( c ) SEC-MALS chromatogram of His-FAK-cTERM-Y925F shows its elution as a single peak of 32±1 kDa. ( d ) SEC-MALS profile of His-CryAB and His-cTERM-Y925F mixture. His-CryAB and His-cTERM-Y925F elute as isolated proteins. The first peak corresponds to His-CryAB (600±5 kDa) and the second to His-cTERM-Y925F (34±1 kDa). ( e ) FAK and pY925-FAK immunoblots of protein extracts from C2C12 cells transfected with pRc/CMV-myc , pRc/CMV-myc-FAK (myc-FAK) or pRc/CMV-myc-FAK-Y925F (myc-FAK-Y925F) vectors. ( f ) Representative ( n =4) anti-αB-crystallin and anti-myc-tag immunoblots of anti-myc-tag immunoprecipitates (IP) from C2C12 cells treated as indicated. Full size image We next substantiated the influence of Y925 on the association of FAK with αB-crystallin in cells. For that, we used FAK expression constructs, one of which harboured myc-tagged FAK (myc-FAK) and the other an Y925F mutant version (myc-FAK-Y925F). These constructs and the empty plasmid (pRc/CMV-myc) were expressed in C2C12 cells ( Fig. 5e ). Precipitates of a myc-specific antibody from C2C12 cells expressing the myc-FAK-Y925F construct contained markedly less αB-crystallin than those obtained from cells expressing myc-FAK ( Fig. 5f ). We also used FLIM-FRET approach to test whether the pharmacological inhibition of Src (PP2) could decrease the association of FAK with αB-crystallin. Single-cell FLIM quantification was carried out before and after (30 min) adding PP2 to the culture medium. PP2 treatment induced a shift in the fluorescence lifetime from 1.8 to 2.4 ns in HEK 293T cells co-expressing the pair CFP-CryAB and YFP-cTERM, but not in cells co-expressing the pair CFP-CryAB and YFP ( τ m =2.4 ns), used as control ( Supplementary Fig. 6d ). In line with this data, we demonstrated an increase in the fluorescence lifetime to 2.3 ns when the pair CFP-CryAB and YFP-cTERM-Y925F was expressed in HEK 293T cells ( Supplementary Fig. 6e ). These results support the notion that Y925 is critical for the interaction between FAK and αB-crystallin in cells. Structural basis of the FAK-cTERM-αB-crystallin interaction To gather information on the structural features of the FAK-cTERM-CryAB complex, we used crosslinking in combination with mass spectrometry (CXMS) analysis and computational modelling [26] , [27] . Given the size and high flexibility of the multidomain full-length FAK, we decided to use the truncated FAK-cTERM in the structural and computational studies. FAK His-cTERM and His-CryAB were expressed and co-purified by affinity and SEC. The disuccinimidyl suberate (DSS)-crosslinked FAK His-cTERM-His-CryAB complex was purified by SEC and identified as shifted bands in an SDS–PAGE analysis ( Fig. 6a ; Supplementary Fig. 7a ). Liquid chromatography–MS/MS analyses ( Supplementary Fig. 7b ) of the DSS-crosslinked His-cTERM-His-CryAB complex indicated that the tryptic peptide 920 SNDKVYENVTGLVKAVIEMSSK 941 is bound by the residue K933 to the K103 of His-CryAB sequence 93 VLGDVIEVHGKHEER 107 ( Fig. 6b,c ; Supplementary Fig. 7c ). K933 is located on the surface of FAK FAT helix 1, while K103 is located on the β5 strand of αB-crystallin. To model the potential interaction site between FAK-cTERM and αB-crystallin, we performed a molecular docking (GRAMM-X protein–protein docking) with the solved structures of FAK FAT (PDB code 1K40) and a Mus musculus model of αB-crystallin ACD (derived from PDB code 2KLR). The docking search was run twice with no search space restriction on the possible docking poses and recovered 300 solutions in each submission. Then, we applied distance restrictions between C-alpha of lysine pair of 20 Å to filter poses into the best energy-ranked solution set. Poses achieved by this approach had lysines 103 and 933 in a position that resembles the DSS-crosslinked lysines. This set of poses was superposed (root mean squared deviation of ~0.5 A) and one model was chosen for the analysis. In this model, the face formed by the α1–α4 helices of FAK FAT interacts with the β4–β8 groove of the ACD ( Fig. 6d ). The structural model of the FAK FAT-αB-crystallin ACD complex was submitted to energy minimization to relieve the problematic van der Waals contacts and to rectify any potentially incorrect geometry that may have existed in the model ( Fig. 6e ). Contact surface analyses showed that this interaction buries an area of ~1,160 A 2 . Importantly, this model can explain the 2:2 stoichiometry of FAK-cTERM:αB-crystallin that emerged from SEC-MALS approach, with one FAK-cTERM monomer able to interact with each copy of the binding site on the opposing faces of the αB-crystallin dimer ( Supplementary Fig. 7d ). 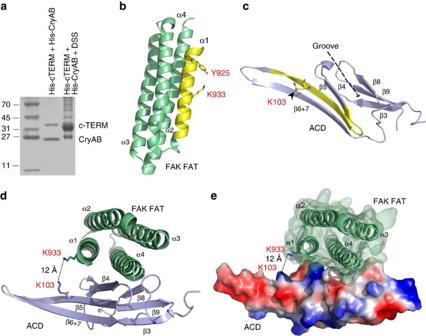Figure 6: FAK FAT domain and αB-crystallin-interacting surface as determined by CXMS and molecular docking. (a) Coomassie blue-stained SDS–PAGE of co-purified His-cTERM-His-CryAB complex and its DSS-crosslinked complex. (b) Ribbon representation of the FAK FAT domain with the crosslinked peptide (SNDKVYENVTGLVKAVIEMSSK) in yellow. The reagent lysine (K933) and the tyrosine 925 are shown in stick representation. (c) Ribbon representation of the ACD of αB-crystallin with the crosslinked peptide (VLGDVIEVHGKHEER) in yellow. The reagent lysine (K103) is arranged near the edge of the hydrophobic binding groove. (d) Ribbon representation of the FAK FAT-α-crystallin (ACD) domain complex. The distance between the lysines crosslinked by the DSS reagent (K933 and K103) is ~12 Å. (e) Surface representation of the FAK FAT-ACD complex (red: negative charges; blue: positive charges; grey: neutral). FAK FAT domain—PDB: 1K40 and ACD model—derived fromPDB: 2KLR. Figure 6: FAK FAT domain and αB-crystallin-interacting surface as determined by CXMS and molecular docking. ( a ) Coomassie blue-stained SDS–PAGE of co-purified His-cTERM-His-CryAB complex and its DSS-crosslinked complex. ( b ) Ribbon representation of the FAK FAT domain with the crosslinked peptide (SNDKVYENVTGLVKAVIEMSSK) in yellow. The reagent lysine (K933) and the tyrosine 925 are shown in stick representation. ( c ) Ribbon representation of the ACD of αB-crystallin with the crosslinked peptide (VLGDVIEVHGKHEER) in yellow. The reagent lysine (K103) is arranged near the edge of the hydrophobic binding groove. ( d ) Ribbon representation of the FAK FAT-α-crystallin (ACD) domain complex. The distance between the lysines crosslinked by the DSS reagent (K933 and K103) is ~12 Å. ( e ) Surface representation of the FAK FAT-ACD complex (red: negative charges; blue: positive charges; grey: neutral). FAK FAT domain—PDB: 1K40 and ACD model—derived fromPDB: 2KLR. Full size image Probing the FAK-cTERM-αB-crystallin complex by mutagenesis To validate the docking model, we performed mutational analysis guided by the predicted interaction regions between FAK-cTERM and αB-crystallin. In addition to Y925F FAK , the FAK-cTERM mutations H1025N FAK , V1029N FAK and L1035N FAK also attenuated this interaction, whereas the mutations V932N FAK , I936N FAK and L1021N FAK did not affect the interaction with CryAB ( Fig. 7a ; Supplementary Fig. 8a ). The CryAB mutation L89N CryAB decreased the interaction, while the mutations V91N CryAB , V93N CryAB and L137N CryAB did not interfere in the interaction with FAK-cTERM ( Fig. 7b ; Supplementary Fig. 8b ). The CryAB combinatorial mutations V91N/V93N CryAB and V91/V93N/L137N CryAB markedly reduced the interaction with FAK-cTERM ( Fig. 7c ; Supplementary Fig. 8b ). 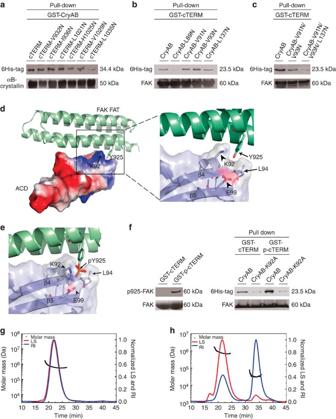Figure 7: Mutagenesis and computational analysis of the FAK-cTERM and CryAB complex interface. (a) Anti-6His-tag and anti-αB-crystallin immunoblots from GST-CryAB pull-down assay performed with FAK His-cTERM and mutants as indicated (n=4). (b,c) Anti-6His-tag and anti-FAK immunoblots from GST-cTERM pull-down assay performed with His-CryAB and mutants as indicated (n=4). (d) FAK FAT-ACD complex model showing the proximity of FAK FAT Y925 (sticks) to the K92 of the ACD. The detailed image shows FAK Y925 docked onto a pocket delimited by K92 and L94 of the β4 strand and E99 of the β5 strand of the ACD. (e) Model showing the rearrangement of α-crystallin K92 towards the phospho-phenolic ring of the Y925-phosphorylated FAK FAT domain. (f) Left panel shows anti-pY925-FAK and anti-FAK immunoblots from GST-cTERM and its Src-phosphorylated form (GST-p-cTERM). Right panel shows representative (n=4) anti-6His-tag and anti-FAK immunoblots from GST-cTERM or GST-p-cTERM pull-down assay performed with His-CryAB and His-CryAB-K92A. (g) SEC-MALS chromatogram of His-CryAB-K92A shows that this protein elutes as a single peak of 640±2 kDa. (h) SEC-MALS profile of His-CryAB-K92A and His-cTERM mixture. His-CryAB-K92A and His-cTERM elute as isolated proteins. The first peak corresponds to His-CryAB-K92A (600±6 kDa) and the second to His-cTERM (32±1 kDa). Figure 7: Mutagenesis and computational analysis of the FAK-cTERM and CryAB complex interface. ( a ) Anti-6His-tag and anti-αB-crystallin immunoblots from GST-CryAB pull-down assay performed with FAK His-cTERM and mutants as indicated ( n =4). ( b , c ) Anti-6His-tag and anti-FAK immunoblots from GST-cTERM pull-down assay performed with His-CryAB and mutants as indicated ( n =4). ( d ) FAK FAT-ACD complex model showing the proximity of FAK FAT Y925 (sticks) to the K92 of the ACD. The detailed image shows FAK Y925 docked onto a pocket delimited by K92 and L94 of the β4 strand and E99 of the β5 strand of the ACD. ( e ) Model showing the rearrangement of α-crystallin K92 towards the phospho-phenolic ring of the Y925-phosphorylated FAK FAT domain. ( f ) Left panel shows anti-pY925-FAK and anti-FAK immunoblots from GST-cTERM and its Src-phosphorylated form (GST-p-cTERM). Right panel shows representative ( n =4) anti-6His-tag and anti-FAK immunoblots from GST-cTERM or GST-p-cTERM pull-down assay performed with His-CryAB and His-CryAB-K92A. ( g ) SEC-MALS chromatogram of His-CryAB-K92A shows that this protein elutes as a single peak of 640±2 kDa. ( h ) SEC-MALS profile of His-CryAB-K92A and His-cTERM mixture. His-CryAB-K92A and His-cTERM elute as isolated proteins. The first peak corresponds to His-CryAB-K92A (600±6 kDa) and the second to His-cTERM (32±1 kDa). Full size image Far-ultraviolet circular dichroism (CD) was used to examine the effects of mutations on the structure of FAK-cTERM and CryAB. CD spectra for FAK-cTERM exhibited two minima (208 and 222 nm), characteristic of α-helix-rich proteins. The mutants Y925F FAK , V932N FAK , I936N FAK , L1021N FAK , H1025N FAK , V1029N FAK and L1035N FAK showed no change in the far-ultraviolet CD ( Supplementary Fig. 8c ). Far-ultraviolet CD spectra for CryAB exhibited single broad ellipticity minima, characteristic of β-sheet and β-turn-rich proteins. The CryAB mutants showed no change in the ellipticity ( Supplementary Fig. 8d ). These analyses indicate that the mutations did not impact the structure of either FAK-cTERM or CryAB proteins. Modelling the enhanced binding of phosphoY925 FAK FAT to ACD The FAK FAT-αB-crystallin ACD complex model revealed that the nonphosphorylated Y925 FAK FAT domain is positioned in close proximity to ACD K92 and is located within a pocket formed by ACD K92 and L94 of the β4 strand and E99 of the β5 strand ( Fig. 7d ). In this configuration, the phenolic moiety of Y925 makes hydrophobic contacts with the aliphatic groups of K92 and L94, and hydrogen bonds with E99 of the β5 strand. Molecular dynamics (MD) simulation (YASARA program) of a Y925-phosphorylated FAK FAT model suggested a rearrangement of the phospho-phenolic ring of Y925 and the positively charged side chain of K92 towards each other and a repulsion of E99 from these contacts ( Fig. 7e ). The MD simulation estimated that Y925 phosphorylation increases the binding free energy by ~122 kcal mol −1 with respect to the nonphosphorylated complex model. Consistent with this model, the CryAB-K92A single mutation markedly decreases the association of CryAB with both the nonphosphorylated and phosphorylated forms of the FAK-cTERM ( Fig. 7f ; Supplementary Fig. 8b ). These results were also validated by SEC-MALS experiments. No change was observed in the elution pattern of CryAB-K92A mutant in comparison with the wild-type CryAB, but the characteristic co-elution peak of the cTERM-CryAB assembly was disrupted ( Fig. 7g,h ). In addition, FRET data obtained with CFP-CryAB-K92A and YFP-cTERM confirmed the lack of interaction between these proteins in the intracellular environment ( Supplementary Fig. 9 ). Together, these results support the notion that FAK binds to αB-crystallin through a specific interaction that is positively modulated by FAK phosphorylation at Y925. αB-crystallin depletion prompts FAK degradation by calpain Given the demonstration that FAK interacts with αB-crystallin in cardiomyocytes subjected to mechanical stress, we asked whether the depletion of αB-crystallin by RNA interference (RNAi; Supplementary Fig. 10a–c ) could influence FAK signalling in cardiomyocytes. We examined FAK protein levels in extracts obtained from non-stretched and stretched cardiomyocytes with an antibody specific to FAK C terminus. A marked reduction of FAK protein level was observed in the stretched, but not in the non-stretched NRVMs that were silenced for αB-crystallin ( Fig. 8a ). This reduction was accompanied by an increase in the cleavage band of ~35 KDa in size when compared with their non-stretched counterparts ( Fig. 8a ). 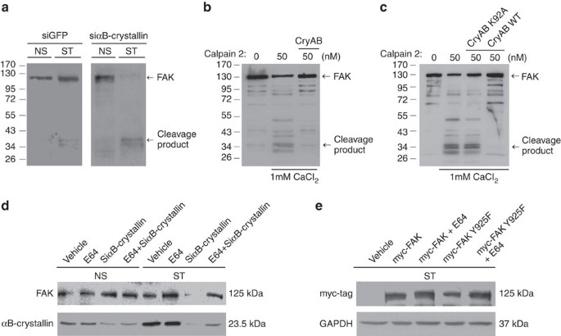Figure 8: Depletion of αB-crystallin downregulates FAK by calpain-mediated proteolysis. (a) Anti-FAK immunoblots of extracts from NS or ST (2 h) NRVMs transfected with RNAi against αB-crystallin (siαB-crystallin) or GFP (siGFP). Shown are FAK (~125 kDa) and its cleavage band (~35 kDa;n=6). (b) Anti-FAK immunoblot fromin vitrocalpain cleavage assay performed with FL-FAK (full-length FAK) and CryAB-WT. The assay was performed by incubating FAK in the cleavage buffer; FAK with calpain 2 and 1 mM CaCl2; and FAK with His-CryAB-WT, calpain 2 and 1 mM CaCl2(n=6). (c) FAK immunoblot fromin vitrocalpain assay performed with FAK and CryAB-K92A. Shown are FAK; FAK with calpain 2 and 1 mM CaCl2; FAK with His-CryAB-K92A, calpain 2 and 1 mM CaCl2; and FAK with His-CryAB-WT, calpain 2 and 1 mM CaCl2(n=6). (d) Attenuation of FAK proteolysis by E64 in NRVMs depleted of αB-crystallin by RNAi. Shown are representative (n=6) anti-FAK and anti-αB-crystallin immunoblots of NS and ST (2 h) NRVMs depleted of αB-crystallin or not, treated with vehicle (Lipofectamine 2000, Invitrogen), or E64. (e) Anti-myc-tag and anti-GAPDH immunoblots of extracts from stretched (2 h) NRVMs transfected with vehicle (Lipofectamine 2000, Invitrogen),pRc/CMV-myc-FAK(myc-FAK),pRc/CMV-myc-FAK+E64,pRc/CMV-myc-FAK-Y925F(myc-FAK-Y925F) or withpRc/CMV-myc-FAK-Y925F+E64 (n=4). GAPDH served as loading control. Figure 8: Depletion of αB-crystallin downregulates FAK by calpain-mediated proteolysis. ( a ) Anti-FAK immunoblots of extracts from NS or ST (2 h) NRVMs transfected with RNAi against αB-crystallin (siαB-crystallin) or GFP (siGFP). Shown are FAK (~125 kDa) and its cleavage band (~35 kDa; n =6). ( b ) Anti-FAK immunoblot from in vitro calpain cleavage assay performed with FL-FAK (full-length FAK) and CryAB-WT. The assay was performed by incubating FAK in the cleavage buffer; FAK with calpain 2 and 1 mM CaCl 2 ; and FAK with His-CryAB-WT, calpain 2 and 1 mM CaCl 2 ( n =6). ( c ) FAK immunoblot from in vitro calpain assay performed with FAK and CryAB-K92A. Shown are FAK; FAK with calpain 2 and 1 mM CaCl 2 ; FAK with His-CryAB-K92A, calpain 2 and 1 mM CaCl 2 ; and FAK with His-CryAB-WT, calpain 2 and 1 mM CaCl 2 ( n =6). ( d ) Attenuation of FAK proteolysis by E64 in NRVMs depleted of αB-crystallin by RNAi. Shown are representative ( n =6) anti-FAK and anti-αB-crystallin immunoblots of NS and ST (2 h) NRVMs depleted of αB-crystallin or not, treated with vehicle (Lipofectamine 2000, Invitrogen), or E64. ( e ) Anti-myc-tag and anti-GAPDH immunoblots of extracts from stretched (2 h) NRVMs transfected with vehicle (Lipofectamine 2000, Invitrogen), pRc/CMV-myc-FAK (myc-FAK), pRc/CMV-myc-FAK +E64, pRc/CMV-myc-FAK-Y925F (myc-FAK-Y925F) or with pRc/CMV-myc-FAK-Y925F +E64 ( n =4). GAPDH served as loading control. Full size image On the basis of previous data [28] , we reasoned that the reduction of FAK in the stretched NRVMs depleted of αB-crystallin could be related to calpain-mediated proteolysis of FAK. To examine this more directly, we tested whether calpain 2 could perform proteolysis on purified recombinant full-length FAK ( Supplementary Fig. 10d ). In fact, in the presence of calcium, calpain 2 displayed significant proteolytic activity towards FAK, as indicated by the reduction of the 125 kDa band and by the generation of the 35 kDa cleavage band of FAK in the in vitro assay ( Fig. 8b ). However, when the solution was first incubated with His-CryAB, we observed a reduction in the FAK cleavage by calpain, indicating that αB-crystallin can function directly to impair the proteolysis of FAK by calpain. To further test this notion, we performed assays with the mutant CryAB-K92A, which is defective in binding FAK. Consistent with the hypothesis that an interaction with αB-crystallin is needed to protect FAK from proteolysis by calpain, the mutant CryAB-K92A was unable to impair FAK degradation by calpain ( Fig. 8c ). We then examined whether the pharmacological inhibition of calpain could influence the FAK protein levels in cardiomyocytes depleted of αB-crystallin. Notably, treatment with the calpain inhibitor E64 abolished the reduction of FAK protein levels in the stretched cardiomyocytes depleted of αB-crystallin ( Fig. 8d ). Further evidence for our model was provided by experiments with cardiomyocytes overexpressing myc-FAK or myc-FAK-Y925F mutant. Western blot performed with anti-myc antibody showed a marked reduction in the amount of myc-FAK-Y925F, but not in myc-FAK, in cardiomyocytes subjected to cyclic stretch. Pretreatment with E64 prevented the reduction of the myc-FAK-Y925F mutant, which is consistent with myc-FAK mutant reduction in stretched cardiomyocytes requiring calpain activity ( Fig. 8e ). These data support the notion that the lack of interaction with αB-crystallin makes FAK susceptible to proteolysis by calpain in the stretched cardiomyocytes. FAK depletion by αB-crystallin silencing elicits apoptosis Since αB-crystallin and FAK may influence the viability and the hypertrophic response of cardiomyocytes to stress [13] , [19] , NRVMs depleted of αB-crystallin were analysed after prolonged (12 h) mechanical stress. Non-stretched cardiomyocytes depleted of αB-crystallin showed a minor reduction in cell viability, but no change in cell morphology ( Fig. 9a ). However, αB-crystallin knockdown led to an enhanced apoptosis and an elongated phenotype, instead of the typical hypertrophy, in stretched cardiomyocytes ( Fig. 9a,b ; Supplementary Fig. 11a ). We next explored whether exogenous expression of myc-FAK might rescue the viability of stretched cardiomyocytes depleted of αB-crystallin. As expected, FAK levels were increased in NRVM cultures transfected with the myc-FAK construct ( Fig. 9c ). The purity of ~97% and the low transfection rate of non-myocytes (<0.02%) in this culture, as estimated by the transfection rates of pEGFP-N1 ( Supplementary Table 2 ), suggest that the cardiomyocytes contribute substantially to the enhanced expression of FAK in cultures transfected with myc-FAK. Notably, the overexpression of a myc-FAK construct rescued the viability of the stretched NRVMs depleted of αB-crystallin ( Fig. 9c ; Supplementary Fig. 11a ), which is consistent with the notion that the reduction of FAK expression is a critical determinant of the reduced viability of stretched cardiomyocyte depleted of αB-crystallin. Additional experiments performed with non-stretched and stretched NRVMs showed that treatment with the calpain inhibitor E64 attenuated the enhanced apoptosis induced by αB-crystallin depletion in stretched NRVMs ( Fig. 9d ; Supplementary Fig. 11a ). These data suggest an important role for the calpain-induced FAK proteolysis in the reduction of the viability of stretched cardiomyocytes depleted of αB-crystallin. 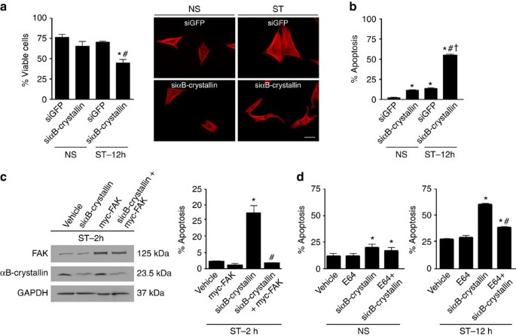Figure 9: Depletion of αB-crystallin prompts mechanically stressed cardiomyocytes to apoptosis. (a) Bar graph represents the quantitative analyses of cell viability (trypan blue viability assay) from NS and ST NRVMs transfected with siGFP or siαB-crystallin. *P<0.0001 versus NS NRVMs transfected with siαB-crystallin.#P<0.0001 versus ST NRVMs transfected with siGFP. Data are presented as mean±s.e.m. (n=6).Pvalues were determined by analysis of variance (ANOVA) and Bonferroni’spost hoccomparisons. Right panel shows immunofluorescence imaging of NS and ST (12 h) NRVMs transfected with siαB-crystallin or siGFP and stained with rhodamine-conjugated phalloidin. Scale bar, 10 μm. (b) Bar graph represents the quantitative analyses of apoptosis (TUNEL assay) performed with NS and ST NRVMs transfected with siGFP or siαB-crystallin. *P<0.0001 versus NS NRVMs transfected with siGFP.#P<0.0001 versus NS NRVMs transfected with siαB-crystallin.†P<0.0001 versus ST NRVMs transfected with siGFP. Data are presented as mean±s.e.m. (n=6).Pvalues were determined by ANOVA and Bonferroni’spost hoccomparisons. (c) Representative (from six independent experiments) anti-FAK, -αB-crystallin and -GAPDH immunoblots of ST (2 h) NRVMs treated with vehicle, transfected with siαB-crystallin, pRc/CMV-myc-FAK (myc-FAK) or pRc/CMV-myc-FAK+siαB-crystallin. Bar graph represents the quantitative analyses of apoptosis from stretched NRVMs treated as indicated. *P<0.0001 versus NRVMs treated with vehicle.#P<0.0001 versus NRVMs transfected with siαB-crystallin. Data are presented as mean±s.e.m.Pvalues were determined by ANOVA and Bonferroni’spost hoccomparisons. (d) Bar graphs represent the quantitative analyses of apoptosis from NS and ST NRVMs treated as indicated (from four independent experiments). *P<0.0001 versus NRVMs treated with vehicle. #P<0.0001 versus ST NRVMs transfected with siαB-crystallin. Data are presented as mean±s.e.m.Pvalues were determined by ANOVA and Bonferroni’spost hoccomparisons. Figure 9: Depletion of αB-crystallin prompts mechanically stressed cardiomyocytes to apoptosis. ( a ) Bar graph represents the quantitative analyses of cell viability (trypan blue viability assay) from NS and ST NRVMs transfected with siGFP or siαB-crystallin. * P <0.0001 versus NS NRVMs transfected with siαB-crystallin. # P <0.0001 versus ST NRVMs transfected with siGFP. Data are presented as mean±s.e.m. ( n =6). P values were determined by analysis of variance (ANOVA) and Bonferroni’s post hoc comparisons. Right panel shows immunofluorescence imaging of NS and ST (12 h) NRVMs transfected with siαB-crystallin or siGFP and stained with rhodamine-conjugated phalloidin. Scale bar, 10 μm. ( b ) Bar graph represents the quantitative analyses of apoptosis (TUNEL assay) performed with NS and ST NRVMs transfected with siGFP or siαB-crystallin. * P <0.0001 versus NS NRVMs transfected with siGFP. # P <0.0001 versus NS NRVMs transfected with siαB-crystallin. † P <0.0001 versus ST NRVMs transfected with siGFP. Data are presented as mean±s.e.m. ( n =6). P values were determined by ANOVA and Bonferroni’s post hoc comparisons. ( c ) Representative (from six independent experiments) anti-FAK, -αB-crystallin and -GAPDH immunoblots of ST (2 h) NRVMs treated with vehicle, transfected with siαB-crystallin, pRc/CMV-myc-FAK (myc-FAK) or pRc/CMV-myc-FAK+siαB-crystallin. Bar graph represents the quantitative analyses of apoptosis from stretched NRVMs treated as indicated. * P <0.0001 versus NRVMs treated with vehicle. # P <0.0001 versus NRVMs transfected with siαB-crystallin. Data are presented as mean±s.e.m. P values were determined by ANOVA and Bonferroni’s post hoc comparisons. ( d ) Bar graphs represent the quantitative analyses of apoptosis from NS and ST NRVMs treated as indicated (from four independent experiments). * P <0.0001 versus NRVMs treated with vehicle. # P <0.0001 versus ST NRVMs transfected with siαB-crystallin. Data are presented as mean±s.e.m. P values were determined by ANOVA and Bonferroni’s post hoc comparisons. Full size image We next examined whether the depletion of myocardial αB-crystallin potentiate the load-induced apoptosis in the left ventricle of TAC mice. To test this, we used RNAi to induce the depletion of myocardial αB-crystallin in mice subjected to a 7-day TAC protocol. αB-crystallin silencing was confirmed by western blot in samples of mice left ventricle ( Supplementary Fig. 11b ). TAC mice depleted of αB-crystallin displayed increased apoptosis of the cardiomyocytes from the left ventricle, as compared with the TAC controls treated with an irrelevant siRNA (siGFP). The basal left ventricular apoptosis was similar between SO mice treated with siRNA targeted to αB-crystallin or with the irrelevant siRNA ( Supplementary Fig. 11c ). We next sought to examine whether FAK expressed in excess would attenuate the enhanced apoptosis in TAC mice depleted of αB-crystallin. To test this, we used a mice model with cardiac-specific transgenic FAK overexpression [17] . αB-crystallin silencing in the heart of transgenic FAK mice was confirmed by western blot ( Supplementary Fig. 11b ). The apoptosis induced by TAC in the transgenic FAK mice silenced for αB-crystallin was reduced by ~50% in comparison with that of the wild-type controls ( Supplementary Fig. 11c ), likely reflecting the protection conferred by FAK. In this study, we revealed a novel interaction between FAK and αB-crystallin mediated by FAK FAT domain that renders FAK less susceptible to proteolytic degradation by calpain. The experiments we report in isolated cardiomyocytes and in the left ventricle of rodents demonstrate that mechanical stress induces a rapid association of active FAK with αB-crystallin. αB-crystallin knockdown sensitizes mechanically stressed cardiomyocytes to calpain-dependent degradation of FAK and to apoptosis. Furthermore, FAK overexpression was shown to be capable of reversing the stretch-dependent apoptosis in cardiomyocytes depleted of αB-crystallin. Thus, the binding of active FAK to αB-crystallin represents a functionally relevant mechanism by which cells such as cardiomyocytes are enabled to cope with the burden of stress and maintain homeostasis. αB-crystallin is proposed to interact with exposed hydrophobic patches of partially unfolded proteins, preventing their aggregation [4] . The results of the in vitro and in vivo experiments presented here provide evidence that αB-crystallin can bind FAK in its folded state. This observation is of interest as emerging data suggest a role for αB-crystallin in binding and regulating folded signalling proteins [14] , [15] . A complete understanding of how an interplay with αB-crystallin results in regulation of FAK function requires knowledge of structural features of the αB-crystallin:FAK complex. In this study, we used protein chemical crosslinking combined with mass spectrometry and mutational analyses [26] , [27] to show that a surface-exposed patch sited between α1 and α4 helices of the FAK FAT domain binds to the β4–β8 hydrophobic groove of ACD. The hydrophobic nature of the FAK FAT α1–α4 patch has been reported to favour its sequestration within intermolecular interfaces of FAK protein partners. For example, this patch binds to paxillin, targeting FAK to focal adhesions in an interaction that has to be disrupted to allow downstream signalling by FAK [29] . Concerning the β4–β8 groove of αB-crystallin, it is key to the cross-binding of the αB-crystallin C-terminal tail in the homodimer interface of the αB-crystallin oligomers [6] , [7] . This suggests that αB-crystallin will not bind FAK efficiently until it is dissociated in suboligomers, when the β4–β8 groove is exposed. An interesting point to this observation is that our SEC-MALS data indicate that the αB-crystallin:FAK FAT domain complex assumes a configuration of a dimer of αB-crystallin bound to two FAK FAT domain monomers. This is consistent with the available structural information regarding αB-crystallin homodimer, which displays the equivalent β4–β8 grooves of each ACD protomer exposed and free to bind to protein partners. An important aspect of our biochemical data and computational model is the crucial contribution of FAK Y925 to the core interaction between the FAK C-terminal domain and a previously unrecognized pocket formed by K92 and L94 at the edge of the αB-crystallin β4 strand. This model provides a mechanistic explanation for the enhanced binding of Y925-phosphorylated FAK C-terminal domain to αB-crystallin. Phosphorylation is predicted to strengthen the binding of the FAK C-terminal domain by repositioning the phenolic side chain of Y925 to within a salt-bridging distance of the positively charged side chain of αB-crystallin K92. These considerations suggest that αB-crystallin recognizes a specific module in the native FAK FAT domain that includes Y925 and other hydrophobic residues. Thus, these data support the concept that αB-crystallin functions not only as a component of the chaperone system but may also bind signalling molecules through specific interactions, clearly illustrating the utility of αB-crystallin as a scaffolding protein. In this context, it is interesting to note that the phosphorylation of FAK Y925 is known to favour an interaction with the adaptor protein Grb2, which has been implicated in the regulation of Erk1/2 pathway [22] . Therefore, it is likely that the interaction with αB-crystallin results in an attenuation of the Erk1/2 activation by FAK, unless the interactions of FAK with Grb2 and αB-crystallin are confined to distinct subcellular compartments. Consistent with this hypothesis, imaging data of the present study indicate that the stress-induced interaction between FAK and αB-crystallin might be restricted to sarcomeres and the perinuclear cytosol. Our results also help underscore the functional relevance of the interaction between FAK and αB-crystallin in the heart. Using cultured cardiomyocytes as a model system, we have demonstrated that the depletion of αB-crystallin results in a significant reduction in FAK protein levels in mechanically stretched cells. Likewise, in mice hearts depleted of αB-crystallin, mechanical stress induced by pressure overload was accompanied by a reduction in FAK protein levels. In addition, our data indicate that the decline in FAK protein levels that accompanies the depletion of αB-crystallin is related to calpain-mediated proteolysis. Therefore, we reason that on the interaction with αB-crystallin, FAK can escape from degradation by calpain, a proteolytic enzyme that is activated and plays an important role in preserving cardiac and skeletal muscle homeostasis in stress conditions [30] . However, the method by which the interaction with αB-crystallin impedes calpain-mediated FAK proteolysis remains unclear. It is notable that calpain cleaves FAK after Ser-745, between the two C-terminal proline-rich regions [28] , which are located in an unstructured region not far from the FAK FAT domain. Thus, we speculate that the interaction of the FAK C-terminal domain with αB-crystallin may somehow impede the access of calpain to the FAK cleavage site. FAK regulates many distinct cellular functions, including migration, proliferation, survival, cell–cell signalling, mechanosensing, cell cycle and gene transcription [31] . Particularly in cardiomyocytes, FAK is activated by stimuli such as mechanical forces, neurohormonal factors and hypoxia to promote hypertrophic growth and survival [32] . Here we present evidence that the interaction with αB-crystallin and the consequent protection of FAK against calpain-induced proteolysis represents a critical event in the survival of cardiomyocytes under mechanical stress. As such, pharmacological inhibition of calpain attenuated FAK degradation and apoptosis in stretched cardiomyocytes that were also depleted of αB-crystallin. Moreover, overexpression of FAK either in cultured cardiomyocytes or in the left ventricle of cardiac-specific FAK transgenic mice blunted the stress-induced apoptosis of cardiomyocytes depleted of αB-crystallin. It is noteworthy that the enhanced interaction between FAK and αB-crystallin may persist unabated up to the advanced stages of pathologic hypertrophy in mice. The consequence of this to the pathophysiology of maladaptive hypertrophy was not explored in the present study, but it could possibly slow the disease progression. In this context, one would expect that the depletion of cardiac αB-crystallin or FAK might predispose to the apoptosis of cardiomyocytes and further deterioration of load-induced pathologic hypertrophy. In fact, the ablation of αB-crystallin in the mice heart has been shown to enhance the maladaptive hypertrophy induced by pressure overload [33] . Similarly, FAK depletion seems to predispose to eccentric hypertrophy and heart failure [34] in response to pressure overload in mice, although it has also been shown by an independent group [18] that depletion of FAK attenuates the load-induced hypertrophy in the mice heart. Furthermore, by identifying the interaction of FAK with αB-crystallin through the FAT domain, our study also provides a rationale for the understanding of the regulation of FAK activity by FRNK (FAK-related nonkinase), a separate protein comprising the C terminus of FAK, which is expressed under certain pathophysiological conditions to act as a dominant negative regulator of FAK activity [35] . We anticipate that an enhanced FRNK expression during stress conditions might compete with FAK for the binding with αB-crystallin, therefore prompting FAK to degradation by calpain, which might negatively impact the viability of cardiomyocytes subjected to mechanical stress. This hypothesis is supported by evidence [36] indicating that overexpression of FRNK results in cardiomyocytes apoptosis. Moreover, mice with cardiac-restricted expression of FRNK exhibit remarkably similar developmental and hypertrophic defects as mice with similar temporal deletion of FAK [34] . Thus, the protection of FAK from calpain-induced cleavage provides a mechanism that enables the cardiomyocytes to survive under stress conditions. Importantly, in addition to mechanical stress, FAK interaction with αB-crystallin was demonstrated to occur in response to oxidative stress, indicating that this mechanism may be relevant to the protection of cardiomyocytes to distinct forms of stress. Relevant to this, calpain is involved in the degradation of unfolded sarcomeric and cytoskeletal proteins of cardiomyocytes in stress conditions and disease states [30] . However, calpain activation may also target signalling molecules, including FAK. It is therefore reasonable to posit that the interaction between FAK and αB-crystallin represents an essential strategy to protect FAK and potentially other signalling molecules during stress conditions in which the activation of calpain is necessary for cardiomyocyte homeostasis. Cultured NRVMs Neonatal male rats (Wistar; 1–2-day old) were handled in compliance with the principles of laboratory animal care formulated by the Institutional Committee for Ethics in Animal Research (State University of Campinas). Each primary culture of NRVMs was prepared using about 70 neonatal rat hearts. After the decapitation, the hearts were rapidly excised, rinsed in cold saline solution and minced coarsely. The myocytes were isolated by digestion with pancreatin and type-2 collagenase and then purified on a discontinuous Percoll gradient, suspended in plating medium containing 10% horse serum, 5% fetal bovine serum and 0.5% penicillin–streptomycin, and plated in type-I collagen Bioflex plates or in Petri plates (25 mm) and incubated for 44 h under 95% air–5% CO 2 . The medium was then replaced by serum-free DMEM and the cells were incubated for 24 h before use [16] . The purity of cardiomyocyte cultures was estimated using 4',6-diamidino-2-phenylindole (DAPI) and anti-α-actinin antibody (1:100) for staining of nuclei and the cardiomyocyte sarcomeres, respectively. The percentage of cardiomyocytes was ~97%. NRVMs cultured in Bioflex plates were stretched in a Flexercell FX-3000 strain unit to 10% of their resting length at a frequency of 1 Hz (0.5 s stretch/0.5 s relaxation) for variable periods of time. At the conclusion of the experimental protocols, cells were scraped from membranes and lysed for immunoblottings or fixed for analysis by fluorescence microscopy. NRVM treatment To obtain myc-FAK or myc-FAK-Y925F overexpression, NRVMs were transfected with 500 ng ml −1 of pRc/CMV-myc-FAK or pRc/CMV-myc-FAK-Y925F constructs. Given that myc and FAK are both expressed as endogenous proteins, we used EGFP construct, DAPI and anti-α-actinin staining to access the efficiency of gene transfer in neonatal cardiomyocytes. We obtained ~20% of transfected NRVMs. To determine whether interaction with αB-crystallin inhibits the cleavage of FAK by calpain, NVMRs were treated with 10 μM of the calpain inhibitor E64 ( N -[ N -( L -3- trans -carboxyirane-2-carbonyl)- L -leucyl]-agmatine; [1-[ N -[( L -3-trans-carboxyoxirane-2-carbonyl)- L -leucyl]amino]-4-guanidinobutane] (Sigma-Aldrich). To deplete αB-crystallin, NRVMs were transfected with 200 ng ml −1 of a specific siRNA using the Lipofectamine 2000 reagent (2 μl ml −1 ; Invitrogen) [37] . NRVMs transfected with siRNA against GFP was used as control. The primers used for the in vitro synthesis of the siRNAs are displayed in Supplementary Table 3 . Isolation of adult rat ventricular myocytes Adult cardiomyocytes were isolated from male Wistar rats (7–8-week old) after SO or TAC (2 h), anaesthetized with a mixture of ketamine (30 mg kg −1 ) and xylazine (5 mg kg −1 ). Cardiomyocytes were isolated by enzymatic dissociation of the whole heart on a Langendorff apparatus. Hearts were excised in ice-cold Tyrode’s solution and perfused retrogradely with the oxygenated solutions: (1) modified Tyrode’s solution containing 1.0 mM Ca 2+ (2 min), (2) Ca 2+ -free Tyrode’s solution (2–3 min), (3) Ca 2+ -free Tyrode’s solution containing 0.2 Wünsch U ml −1 of collagenase (Sigma, USA) for 20 min and (4) followed by washing in Kruftbrühe (KB) solution for 5 min. Digested atrium and ventricles were cut off and minced in KB solution, pipetting to dissociate the cells, then filtered through a nylon mesh (200 μm pore size) to remove big pieces of undigested tissues. Isolated cells were rinsed in KB solution and allowed to settle by gravity three times to remove debris and non-cardiomyocytes. Resuspended cells in KB solution were loaded above the top layer of a Percoll gradient formed by 20%, 40% and 70% Percoll and centrifuged at 100 g for 20 min to further purify cardiomyocytes. Purified myocytes after Percoll gradient separation were homogenized in lysis buffer and used in western blotting and immunoprecipitation protocols. Modified Tyrode’s solution contained: 10 mM HEPES, 105 mM NaCl, 0.6 mM KH 2 PO 4 , 5.4 mM KCl, 6 mM NaHCO 3 , 0.6 mM NaH 2 PO 4 , 1 mM MgCl 2 , 5 mM KHCO 3 , 1 mM CaCl 2 , 20 mM taurine and 5 mM glucose (pH 7.35—NaOH), and KB solution: 10 mM HEPES, 20 mM KCl, 1 mM MgCl 2 , 70 mM K + -glutamate, 10 mM KH 2 PO 4 , 25 mM glucose, 20 mM taurine, 10 mM b-hydroxybutyric acid, 0.1% albumin and 0.5 mM EGTA (pH 7.25—KOH) [38] . Mice Swiss mice (6–8-week old) were handled in compliance with the principles of laboratory animal care formulated by the Animal Care and Use Committee of the State University of Campinas. Procedures such as jugular vein catheterization, aortic banding, echocardiographic examination and arterial vessel catheterization for blood pressure monitoring were performed under anaesthesia with a mixture of ketamine (100 mg kg −1 ) and xylazine (5 mg kg −1 ). Aortic banding was performed by TAC by tying a 7-0 nylon (Dafilon; B.Braun Melsungen AG, Germany) suture ligature against a 27-gauge needle. SO animals were prepared in the same way, except for the aortic constriction. For the blood pressure monitoring, the right carotid and the right femoral arteries were cannulated with flame-stretched PE-50 polyethylene tube. Blood pressure in the carotid and femoral arteries was simultaneously recorded for a 10-min period to determine the transconstriction systolic gradient. The recordings were obtained from a COBE transducer (Arvada, USA), connected to a GP4A Stemtech amplifier (Stemtech, USA). The amplifier output was connected to an analogue-to-digital board and this to a computer loaded with WINDAQ-PRO Data Acquisition software (DATAQ Instruments, USA), for continuous blood pressure monitoring. Pulsatile blood pressure from carotid and femoral catheters was recorded in individual channels and sampled at 100-Hz [39] , [40] . Immunoprecipitation NRVMs or tissues homogenized in lysis buffer were normalized (500 μg) and incubated with anti-αB-crystallin polyclonal (2 μg; Santa Cruz Biotechnology), anti-myc-tag monoclonal (2 μg; Sigma-Aldrich) or with anti-FAK-c20 (2 μg; Santa Cruz Biotechnology) polyclonal antibodies. The proteins were collected after addition of 20 μl of protein A-sepharose beads (GE Healthcare). Western blots of the immunoprecipitates were performed with anti-FAK-c20 (1:1,000; Santa Cruz Biotechnology), anti-p397FAK (1:1,000; Invitrogen), anti-p925FAK (1:1,000; Santa Cruz Biotechnology), anti-αB-crystallin (1:1,000; Santa Cruz Biotechnology) or anti-myc (1:2,500; Sigma-Aldrich) antibodies. Quantification of bands was performed using Image J (Image Processing and Analysis in JAVA-program/National Institutes of Health NIH). The uncropped blots are displayed in Supplementary Fig. 12 . Microscopy analysis Fixed cells or tissues were blocked with 1% bovine serum albumin, 0.1% Triton-X and 50 nM glycine in 0.1 M phosphate-buffered saline (PBS) on ice. Then, samples were incubated with anti-FAK c-20 (1:100) and subsequently with anti-αB-crystallin (1:100) antibody overnight at 4 °C. Next, Alexa Fluor-488-conjugated goat anti-rabbit (1:200) and Alexa Fluor-568-conjugated goat anti-mouse (1:200) secondary were used at room temperature, followed by Alexa Fluor-647 phalloidin (1:50; Invitrogen). Alternatively, NRVMs were incubated with rhodamine-conjugated phalloidin (1:50; Molecular Probes) at room temperature for 2 h. Slides were then mounted with VectaShield with DAPI. Confocal images were obtained with a LEICA TCS SP8 microscope. Fluorescence images were obtained with a LEICA DM4000 fluorescence microscope. Protein cloning and purification The pGEX2T constructs encoding the GST FERM (GST-FERM; ~70 kDa), GST-Kinase (~55 kDa) and GST-FAK C terminus (GST-cTERM; ~60 kDa) fusion proteins were described previously [26] . The GST-CryAB construct (1–175 aa; ~49.5 kDa) encoding the full-length protein αB-crystallin was cloned in the BamHI site of pGEX2T . 6xHis-tagged αB-crystallin (His-CryAB) was obtained by cloning the αB-crystallin sequence between the NdeI and XhoI sites of pET-15b (1–175 aa; ~23 kDa), while the His-cTERM construct was obtained by cloning its sequence into the NdeI and BamHI sites of pET-15b (765–1,052 aa; ~34 kDa). The cloning primers are listed in Supplementary Table 3 . Plasmid encoding the c-Src kinase domain containing a YopH phosphatase was provided by Dr John Kuriyan. Plasmid encoding the wild-type myc-FAK construction ( pRc/CMV-myc-FAK ) was provided by Dr Steven K. Hanks and its mutated form was obtained by site-directed mutagenesis. The 6xHis-tagged constructions were expressed in E. coli Bl21 (DE3) C41 cells and purified by affinity chromatography (HisTrap HP 5 ml, GE Healthcare Bio-Sciences, Piscataway, NJ, USA). Next, an ion exchange chromatography was performed using buffer A—50 mM Tris, pH 7.5, 50 mM NaCl—and buffer B—50 mM Tris, pH 7.5, 1 M NaCl (HiTrap Q HP and HiTrap SP HP, GE Healthcare)—followed by a SEC in 50 mM Tris-HCl, pH 7.5, 150 mM NaCl and 10% glycerol (HiLoad 16/60 Superdex 200 pg, GE Healthcare). The His-cTERM-His-CryAB complex was obtained by incubation of the previously purified His-cTERM and His-CryAB (1:1 molar; overnight; 4 °C) followed by SEC in 50 mM phosphate, pH 7.5, and 150 mM NaCl buffer (HiLoad 16/60 Superdex 200 pg, GE Healthcare). The elution peak containing the co-purified complex was isolated and used to the cross-linking experiments. See also Supplementary Information for full-length FAK purification. Pull-down assay His-CryAB coupled to Ni 2+ sepharose beads was incubated with full-length recombinant human GST-FAK (FL-FAK; Invitrogen, USA) and total extracts from non-stretched (NS) or stretched (ST) NRVMs, as indicated (see Results). GST-FERM, GST-KINASE, GST-cTERM and GST coupled to glutathione sepharose beads were incubated with His-CryAB or total extracts from NS or ST NRVMs. GST-CryAB coupled to glutathione sepharose beads was incubated with His-cTERM plus Src, His-cTERM plus Src and ATP or with His-cTERM-Y925F plus Src and ATP. GST-cTERM coupled to glutathione sepharose beads was incubated with His-CryAB or His-CryAB mutants. The precipitated pellets from the various assays were resolved by SDS–PAGE and the membranes immunoblotted with anti-αB-crystallin (1:1,000; Santa Cruz Biotechnology), anti-FAKc20 (1:1,000; Santa Cruz Biotechnology) or anti-6his-tag (1:2,500; Abcam) antibodies. SEC-MALS The oligomeric state of His-CryAB and His-FAK-cTERM in solution was analysed by SEC-MALS. The measurements were performed on ÄKTA FPLC system (GE Healthcare) connected to a triple-angle static light-scattering detector miniDAWN TREOS and a refractive index detector Optlab-TrEX (Wyatt Technology, Santa Barbara, CA, USA). Purified proteins (1.5 mg ml −1 ; 500 μl) were applied to a Superdex200 HR 10/30 column (GE Healthcare) with a flow rate of 0.5 ml min −1 . Refractive index and light scattering were measured and the data were analysed using ASTRA 6 software after calibration with a bovine serum albumin standard. FRET-FLIM The pAmCyan1-C1 and pZsYellow1-C1 vectors were acquired from Clontech Laboratories. CFP was linked to YFP through a 15-aa-long linker (CFP-15aa-YFP) by inserting the YFP sequence between the SalI and BamHI sites of the pAmCyan1-C1 vector. The CFP-CryAB (wild-type or K92A) and YFP-cTERM (wild-type or Y925F) constructs were generated by subcloning their sequences into the BamHI site of the pAmCyan1-C1 and the pZsYellow1-C1 vectors, respectively. The primers used in cloning reactions are listed in Supplementary Table 3 . The confocal and FLIM images of HEK 293T cells expressing diverse combinations of constructs were acquired with a Zeiss LSM780-NLO microscope (Carl Zeiss AG, Germany). The fluorescence signal was excited with a Mai-Tai laser (Newport, USA) or with an argon laser (Lasos, Germany). The laser was focused by an EC Plan-Neofluar × 40/1.30 Oil DIC, and the same objective collected the signal. The confocal images were acquired with the internal detectors, while the FLIM images were detected with a Hybrid-PMT in the non-descanned port. The FLIM system is composed of a hybrid-PMT, TCSPC cards and a controller computer (all obtained from Becker&Hickl, Germany). CFP was excited at 800 nm and YFP was excited at 488 nm. A short-pass filter at 470 nm was used to reject any YFP fluorescence originating from the excitation at 800 nm. In vitro Src-mediated phosphorylation of FAK C terminus FAK-cTERM and FAK-cTERM-Y925F were dialyzed into phosphorylation buffer (50 mM HEPES, pH 7.0, 30 mM MgCl 2 , 1 mM dithiothreitol, 10% glycerol, 6 mM EGTA, 10 mM sodium orthovanadate and 10 mM sodium tartrate) and incubated with Src and ATP (1 mM) at 30 °C for 90 min. The samples were analysed by MS/MS or incubated with SDS Laemmli sample buffer for western blotting with a phosphospecific antibody. Site-directed mutagenesis The Stratagene QuikChange II XL Site-Directed Mutagenesis Kit was used to produce the myc-FAK, FAK-cTERM domain and the CryAB mutants using the mutagenic primers listed in Supplementary Table 3 . DNA samples from the plasmids pRc/CMV-Myc-FAK , pET15b-cTERM and pET15b-CryAB were used as templates. The mutations were confirmed by DNA sequencing. CXMS The co-purified His-cTERM-His-CryAB complex in 50 mM phosphate buffer, pH 7.5, and 150 mM NaCl was incubated with DSS (disuccinimidyl suberate; suberic acid bis; Sigma-Aldrich) dissolved in dry dimethylformamide in a final 1:100 protein/DSS ratio for 2 h at room temperature [26] , which was followed by quenching with 50 mM Tris buffer, pH 7.6. The proteins were reduced (5 mM dithiothreitol, 25 min at 56 °C), alkylated (14 mM iodoacetamide, 30 min at room temperature in the dark) and digested with trypsin (Promega). The samples were dried in a vacuum concentrator and reconstituted in 100 μl of 0.1% formic acid. The digested sample was fractionated by using Oasis SPE cartridges (Waters) in elution steps of 5, 10, 15, 20, 25 and 70% acetonitrile aqueous solution. Each fraction was dried in evaporator for a final volume of 10 μl and analysed by liquid chromatography–MS/MS performed using a Synapt mass spectrometer (Waters). For chromatography, solvent A was 0.1% aqueous formic acid and solvent B acetonitrile with 0.1% of formic acid. The gradient started with 3% solvent B, increasing linearly to 30 over 40 min, going to 70% for 10 min and going back to 3% after 55 min. The MS/MS data were acquired selecting the top three precursors with 1 s MS/MS acquisition time, selecting precursor ions of charge >2+. The raw data were processed using Mascot Distiller 2.4.3 (Matrix Science) and the processed spectra were used for crosslinked peptide identification using Crux search for xlinks [41] and XLinker Identifier [42] softwares. Crosslinked identification was performed using the following parameters: 0.1 Da tolerance for both MS and MS/MS, hydrolysed DSS for lysines and oxidation for methionine as variable modifications, iodoacetamide as fixed modification on cysteines and three missed cleavages, trypsin digestion. Manual validations of crosslinking assignment were performed on singly charged deconvoluted spectrum. Molecular modelling, docking and dynamics simulation The structure of ACD of Homo sapiens (PDB: 2KLR) was used as a template for the molecular modelling of the Mus musculus ACD (YASARA program). Molecular docking was conducted with the FAK FAT domain of Mus musculus (PDB: 1K40) and the α-crystallin model using the GRAMM-X web server for the molecular docking. To select the most appropriate solution from all the resulting docked conformations, a discrimination procedure based on the CXMS data was applied. The representative model for the complex between FAK FAT and ACD was selected, and submitted to energy minimization and MD simulation using YASARA. For that, all hydrogen atoms and other missing atoms from the model were created using force field parameters obtained from YAMBER3. A simulation box was defined at 15 Å around all atoms of each complex. Protonation was performed based on the pH 7.5. Cell neutralization was reached filling the box with water molecules and Na/Cl counter ions. A short MD was performed for the solvent adjustment, deleting water until the density of 0.997 g ml −1 . A short steepest descent energy minimization was carried out until the maximum atom speed dropped below 2,200 m s −1 . Then, 500 steps of simulated annealing were performed with a temperature of 0 K. Finally, we performed an 8 ns simulation at 298 K and a non-bonded cutoff of 7.86 A. A snapshot was saved every 25 ps. Simulation time was adjusted to stabilize the contacts between proteins. In vitro calpain cleavage assay Recombinant FAK (1 μg) was incubated in cleavage buffer (50 mM Tris-HCl, pH 7.4, 137 mM KCl and 1 mM MgCl 2 ) with 50 nM purified recombinant calpain 2 (Calbiochem) plus 1 mM CaCl 2 at 30 °C for 30 min in the absence or presence of His-CryAB or His-CryAB-K92A (1:1 molar). The cleavage reactions were stopped by addition of 5 × SDS Laemmli sample buffer. Cardiomyocyte viability Non-stretched or stretched NRVMs transfected with siRNA against GFP or αB-crystallin were washed with PBS (pH 7.4), trypsinized for 5 min and centrifuged (12,000 g ). The supernatant was aspirated and the cardiomyocytes were resuspended in a suitable volume of PBS (1 ml) with 0.8% trypan blue. Then, the cells were counted in a Neubauer chamber. The number of dead cells (blue cells—Trypan (+)) in a total of 300 cells was counted in each experiment. Viable cells were represented as the mean percentage of dead cells per total cells [43] . TUNEL assay Apoptotic nuclei of non-stretched or stretched cardiomyocytes treated with E64, RNAi or overexpression assays, or the myocardium of wild-type or FAK transgenic mice were assessed using In Situ Cell Death Detection Kit (Roche). Fixed cells or deparaffinized myocardial sections were washed with PBS and incubated with Proteinase K 20 μg ml −1 for 10 min at 25 °C. For the myocardium, the endogenous peroxidase activity was inhibited using 3% hydrogen peroxide. Subsequently, cells or the myocardium were incubated with TUNEL reaction mixture containing terminal deoxy-nucleotidyl transferase and fluorescein-dUTP for 1 h at 37 °C. For positive control, samples were incubated with DNAse I before the addition of the TUNEL reaction mixture. For negative control, samples were incubated only with fluorescein-dUTP. Cells were mounted with Vectashield with DAPI and then examined by fluorescence microscope [43] . Heart tissues were incubated with substrate mixture of 0.5 mg ml −1 3,3'-diaminobenzidine (Sigma, St Louis, MO, USA) and 0.3% hydrogen peroxide, according to manufacturer’s instruction. The sections were counterstained with Harris haematoxylin and then examined by light microscope. Statistical analyses Analysis of variance and Bonferroni’s post hoc comparisons were used to compare the actual densitometric data from the immunoblots or the quantification of cell viability or apoptosis in the respective experimental groups. P <0.05 was considered to be statistically significant. The data are presented as the mean±s.e.m. for the indicated number of experiments. When presenting the data, we normalized the densitometric values and defined the mean for the control group as 100. How to cite this article: Pereira, M. B. M. et al. αB-crystallin interacts with and prevents stress-activated proteolysis of focal adhesion kinase by calpain in cardiomyocytes. Nat. Commun. 5:5159 doi: 10.1038/ncomms6159 (2014).